Generalized self-assembly of scalable two-dimensional transition metal oxide nanosheets Two-dimensional (2D) transition metal oxide systems present exotic electronic properties and high specific surface areas, and also demonstrate promising applications ranging from electronics to energy storage. Yet, in contrast to other types of nanostructures, the question as to whether we could assemble 2D nanomaterials with an atomic thickness from molecules in a general way, which may give them some interesting properties such as those of graphene, still remains unresolved. Herein, we report a generalized and fundamental approach to molecular self-assembly synthesis of ultrathin 2D nanosheets of transition metal oxides by rationally employing lamellar reverse micelles. It is worth emphasizing that the synthesized crystallized ultrathin transition metal oxide nanosheets possess confined thickness, high specific surface area and chemically reactive facets, so that they could have promising applications in nanostructured electronics, photonics, sensors, and energy conversion and storage devices. Ultrathin two-dimensional (2D) nanostructures are highly desirable for obtaining superior catalytic, photovoltaic and electrochemical performances, due to their large surface-to-volume ratio and confined thickness on the atomic scale [1] , [2] , [3] , [4] , [5] , [6] , [7] , [8] . For example, the 2D carbon network—graphene—features extremely high carrier mobility, mechanical flexibility, optical transparency and chemical stability, which provide a great opportunity for developing new electronic materials, novel sensors and metrology facilities, and superior energy conversion and storage devices [4] , [5] , [6] . Although transition metal oxides have been widely studied as functional materials so far, they are mainly obtained in the form of 0D (nanodots and fine nanoparticles), 1D (nanowires and nanotubes) and 3D mesoporous structures and nanoclusters [9] , [10] , [11] , [12] . In contrast, 2D nanomaterials, especially those with confined thickness, have remained conspicuously absent until the recent emergence of delamination of layered compounds into single layers, referred to as exfoliation or top–down synthesis [3] , [7] , [8] , [13] , [14] , [15] , [16] , [17] , [18] . Only a few 2D metal oxides that have suitably layered host crystals, unfortunately, in which 2D platelets are weakly stacked to form 3D bulk materials, can be obtained via the exfoliation method [3] , [15] , [16] , [17] , [18] . Moreover, the preparation of homogeneous 2D nanosheets on a large scale by exfoliation is also a big challenge. Thus, a generalized bottom-up strategy for controlled synthesis of metal oxides in 2D nanostructures from precise molecular self-assembly is extremely desirable to meet the growing demand for such 2D metal oxides in various applications related to sensing, catalysis, energy storage and electronic devices. Moreover, the bottom-up wet chemistry synthesis of 2D metal oxide nanosheets can meet the demand for homogeneous production on a large scale for practical applications. Thus, a novel synthesis strategy that has flexible capabilities for 2D nanostructure fabrication would be a great breakthrough in nanotechnology, allowing us to take advantage of the high specific surface area, confined atomic level thickness and salient surface chemical states, as well as possible unique mechanical, thermal, electronic and optical properties of the 2D nanostructured metal oxides. Herein, we provided a generalized synthesis strategy for surfactant self-assembly or bottom-up growth of various ultrathin 2D transition metal oxide nanostructures from molecular precursors, in which amphiphilic block copolymers and short-chain alcohol co-surfactants are intelligently employed as structure-directing agents to confine the stacking and growth of the metal oxide along the chosen direction. Surfactant self-assembly has been successfully employed in the synthesis of 0D, 1D and 3D metal oxide nanostructures or mesoporous structures; however, the synthesis of 2D metal oxides still lacks systematic studies [19] , [20] , [21] , [22] , [23] . Our concept for surfactant self-assembly of ultrathin 2D metal oxide nanosheets, as shown in Fig. 1 , is to form inverse lamellar micelles of polyethylene oxide–polypropylene oxide–polyethylene oxide (PEO 20 –PPO 70 –PEO 20 , Pluronic P123) surfactant together with ethylene glycol (EG) co-surfactant in ethanol solvent. The hydrated inorganic oligomers are then confined inside the inverse lamellar micelles, leading to the formation of layered inorganic oligomer agglomerates. In this step, the water content that is used to form the hydrated precursor oligomers is controlled in the phase area to form inverse lamellar micelles based on the phase behaviour of the surfactant–water–oil equilibrium system ( Supplementary Fig. 1 ) [24] , [25] . It has been reported that EG can work in the role of both co-surfactant and co-solvent in the surfactant–water system [26] . Here, the addition of EG is very crucial in the formation of ultrathin 2D metal oxide nanosheets, as it can lead to a more stable lamellar phase compared with the binary surfactant–water system [25] , [26] . Hydrothermal or solvothermal treatment is then carried out to improve the organization and induce complete condensation and crystallization. Finally, well-crystallized ultrathin 2D transition metal oxide nanosheets are collected after the removal of the surfactant templates. Compared with exfoliation synthesis, the biggest merits are that the self-assembly synthesis of metal oxide nanosheets is not restricted by the limited numbers of layered host materials, and synthesis of homogeneous nanomaterials in large quantities is possible. Surfactant self-assembly thus can provide a flexible and general way to synthesize 2D metal oxide nanostructures. This synthesis procedure is successfully applied to the preparation of 2D nanostructures of some typical transition metal oxides such as TiO 2 , ZnO, Co 3 O 4 , WO 3 , Fe 3 O 4 and MnO 2 . 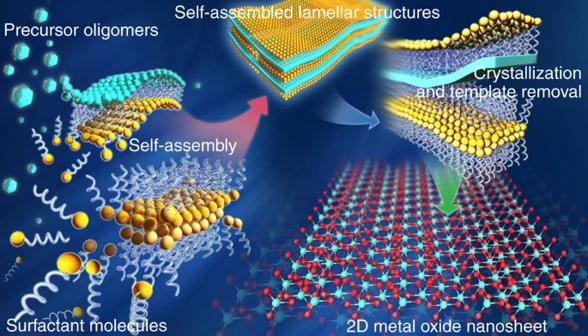Figure 1: Schematic drawing of self-assembly of 2D metal oxide nanosheets. The schematic shows the concept of molecular assembly of ultrathin 2D metal oxide nanosheets from liquid solutions, where metal oxide precursor oligomers are strategically and collaboratively self-assembled into lamellar structures with polymer surfactant molecules, before they are condensed, polymerized and crystallized into 2D metal oxide nanosheets with atomic thickness. Figure 1: Schematic drawing of self-assembly of 2D metal oxide nanosheets. The schematic shows the concept of molecular assembly of ultrathin 2D metal oxide nanosheets from liquid solutions, where metal oxide precursor oligomers are strategically and collaboratively self-assembled into lamellar structures with polymer surfactant molecules, before they are condensed, polymerized and crystallized into 2D metal oxide nanosheets with atomic thickness. Full size image Synthesis and microscopy characterizations of 2D nanosheets In a typical synthesis protocol, Pluronic P123 was dissolved in ethanol to form a transparent surfactant solution. To this solution, metal alkoxides or inorganic metal salts in the desired molar ratio were added under vigorous stirring. The resulting sol solution was then mixed with EG. Solvothermal treatment was then carried out on the as-prepared or the well-aged solutions to form crystallized metal oxide 2D nanosheets. Via this synthesis strategy, ultrathin 2D nanostructures of the typical transition metal oxides, such as TiO 2 , ZnO, Co 3 O 4 , WO 3 , Fe 3 O 4 and MnO 2 , were successfully synthesized. Details of the synthesis procedure for the individual samples can be found in the Methods section and the Supplementary Information . We performed scanning electron microscopy (SEM) and transmission electron microscopy (TEM) analyses on the synthesized ultrathin 2D metal oxide nanostructures. The ultrathin 2D nanosheets of TiO 2 , ZnO, Co 3 O 4 and WO 3 are shown in Fig. 2 . These nanosheets can be clearly distinguished in low-magnification SEM images ( Fig. 2a,d,g,j ) and low-magnification TEM images ( Fig. 2b,e,h,k ). They exist in the form of groups of nanosheets. More detailed electron microscopy characterizations of these ultrathin 2D nanosheets can also be found in Supplementary Figs 2–5 . From these microscope images, it can be seen that the products are all nanosheets with their edges rolled up due to surface tension, which is similar to the general behaviour of graphene. The sizes of the nanosheets vary with the chemical composition: around 200 nm for TiO 2 and 1–10 μm for ZnO, Co 3 O 4 and WO 3 . In addition, the TiO 2 , ZnO, Co 3 O 4 and WO 3 nanosheets present well-crystallized anatase, wurtzite, cubic and monoclinic phase, respectively, as demonstrated by the high-resolution TEM (HRTEM) characterizations (insets in Fig. 2c,f,i,l ) and the corresponding X-ray diffraction (XRD) patterns ( Supplementary Fig. 6 ). The electron microscope characterizations of the ultrathin 2D Fe 3 O 4 and MnO 2 nanosheets are shown in Supplementary Figs 7 and 8 , where the features of the 2D nanosheets are also clearly exhibited. Supplementary Fig. 9 presents the corresponding XRD patterns, approving their characteristics of crystalline. The uniform morphologies of all the obtained ultrathin 2D transition metal oxide nanosheets demonstrate the general and effective nature of the proposed synthesis method, and indicate its feasibility to be extended to the synthesis of other 2D nanostructures. 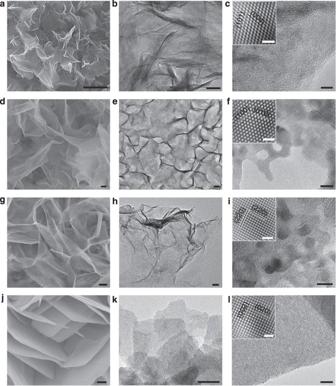Figure 2: Electron microscope images of 2D transition metal oxide nanosheets. SEM images (a,d,g,j), low-magnification TEM images (b,e,h,k) and high-magnification TEM images (c,f,i,l) of ultrathin 2D nanosheets of TiO2(a–c), ZnO (d–f), Co3O4(g–i) and WO3(j–l). The insets inc,f,iandlare high-resolution TEM images of the crystal lattice structure of the nanosheets. Scale bar, 200 nm (a,d,g,j), 50 nm (b,e,h), 20 nm (k), 5 nm (c,f,i,l) and 1 nm (insets inc,f,i,l). Figure 2: Electron microscope images of 2D transition metal oxide nanosheets. SEM images ( a , d , g , j ), low-magnification TEM images ( b , e , h , k ) and high-magnification TEM images ( c , f , i , l ) of ultrathin 2D nanosheets of TiO 2 ( a – c ), ZnO ( d – f ), Co 3 O 4 ( g – i ) and WO 3 ( j – l ). The insets in c , f , i and l are high-resolution TEM images of the crystal lattice structure of the nanosheets. Scale bar, 200 nm ( a , d , g , j ), 50 nm ( b , e , h ), 20 nm ( k ), 5 nm ( c , f , i , l ) and 1 nm (insets in c , f , i , l ). Full size image The thickness of the synthesized ultrathin 2D metal oxide nanosheets was determined based on the conventional used methods employing the TEM and atomic force microscopy (AFM) techniques ( Supplementary Figs 10 and 11 ) [27] , [28] . For TiO 2 nanosheets, as shown in Supplementary Fig. 10 , it was determined that the monolayer thickness of the self-assembled TiO 2 nanosheets is around 0.62 nm by observing the edge configuration. The ultrathin TiO 2 nanosheets synthesized by the present method have a thickness of around 3.3 nm, which implies that they are stacks consisting of 4–5 monolayers. The thickness of the ZnO, Co 3 O 4 and WO 3 ultrathin 2D nanosheets were also determined by AFM ( Supplementary Fig. 11 ). The thicknesses of these metal oxide nanosheets varied between 1.6 and 5.2 nm, corresponding to 2–7 stacking layers of the monolayer ( Supplementary Table 1 ). In general, all the thicknesses of these 2D nanosheets are thin enough to present quantum confinement effects ( Supplementary Fig. 12 ), demonstrating their potential applications in some novel electronic devices. The roles of the added P123 surfactant, EG and water in the formation of the ultrathin 2D nanosheets were investigated by performing the synthesis without one chemical or by changing the amount to be added. Supplementary Fig. 13 presents the morphologies of the nanostructures of TiO 2 ( Supplementary Fig. 13a,c,e,g ) and ZnO ( Supplementary Fig. 13b,d,f,h ) that were synthesized from the solutions: (I) without the addition of P123 ( Supplementary Fig. 13a,b ), (II) without the addition of EG ( Supplementary Fig. 13c,d ), (III) with the addition of 300 wt.% water ( Supplementary Fig. 13e,f ) and (IV) with the addition of 700 wt.% water ( Supplementary Fig. 13g,h ). The morphologies of the nanostructures with modified recipes showed huge deviation from that of the 2D nanosheets. Without P123, even though the 2D morphology is still present in disguised form, the products are mainly in the form of large agglomerates, indicating that the P123 might be absorbed on the surface of the oligomers to resist the contact and growth of 2D nanosheets in a thin dimension. Without EG, almost no nanosheets can be found, demonstrating the key role of EG in the formation of inverse micelles as co-surfactant and co-solvent. EG presents similar behaviour to that of water for non-ionic surfactants in the role of co-solvent. In addition, EG that behaves as co-surfactant facilitates the separation of lamellar phase, leading to the formation of more stable lamellar structures [25] , [26] . In the present study, therefore, the formation of ultrathin 2D transition metal oxide nanosheets should be resulted from a synergetic effect of P123 and EG. The synergetic effect of water-soluble short-chain alcohol and water has been well studied [25] , [26] . It is suggested that utilizing the synergetic effect of the alcohol and surfactant should be effective in constructing desirable aggregate architectures in water–alcohol–surfactant system via adjusting the ratios of alcohol/surfactant, alcohol/water or alcohol/alcohol [25] . Obviously, the role of each chemical is very crucial in the synthesis of 2D nanosheets. Even a small change in the chemical contents of the solution could result in a large deviation from the desirable area in the phase diagram. Surface properties of 2D nanosheets Unlike the bulk crystals, the ultrathin metal oxide nanosheets have an extremely high percentage of surface (nearly 100%). It has been reported that the exposed surfaces present different chemical states from the inner bulk atoms [29] , [30] . The surface chemical states of the ultrathin metal oxide nanosheets were examined by the X-ray photoelectron spectroscopy (XPS) technique ( Fig. 3a–d and Supplementary Table 2 ). It is of interest that the core levels of the metal elements, Ti 2 p , Zn 2 p , Co 2 p and W 4 f , all show a 0.5–2 eV shift to lower binding energy compared with the corresponding stoichiometric bulk crystals [29] , [30] . The lower binding energy for surface atoms has been reported to be the result of electron gain (reduction) of metal atoms from surrounding oxygen atoms, for example, from the Ti 4+ to the Ti 3+ state [30] . We suspect that the chemical state shifting of the transition metal atoms, or the electron transfer from O atoms to metal atoms, probably has resulted from the dramatic distortion of the crystal structure that occurs in the surface-dominated ultrathin metal oxide nanosheets [28] . To clarify this, density functional theory (DFT) calculations were employed to analyse the crystal structure distortion and the electronic density distributions in the free-standing ultrathin 2D metal oxide nanosheets and the corresponding bulk inner atoms, respectively ( Fig. 3e–l ). To give a quantitative estimation of the electron transfer between the metal and oxygen atoms, Löwdin atomic population analysis was also performed for the 2D nanosheets and bulk materials ( Table 1 ). Population analysis is the study of charge distribution and electron transfer within molecules. The intention is to accurately model partial charge magnitude and location within a molecule [31] , [32] , [33] . The DFT calculations reveal that the metal atoms in the ultrathin 2D nanosheets have higher surrounded electron densities that resulted in reduction states compared with the corresponding bulk materials, accompanying with new bond formation, bond breaking or bond distortion between the metal–oxygen atoms of the crystal structures, which coincides well with the XPS chemical state shifts. Therefore, compared with the corresponding inner atomic planes of the bulk materials, the 2D nanosheets present significant lattice distortion and extra chemical bond formation, breaking and distortion, which accompany the redistribution of electron density and significantly less electron transfer from metal atoms to O atoms, which, in turn, results in reduced chemical states of the transition metal atoms in the 2D metal oxide nanosheets. These results demonstrate the unique chemical states of the surface atoms in the ultrathin 2D metal oxide nanosheets, which will introduce some anticipated physical and chemical properties that differ from those associated with the conventional morphologies. 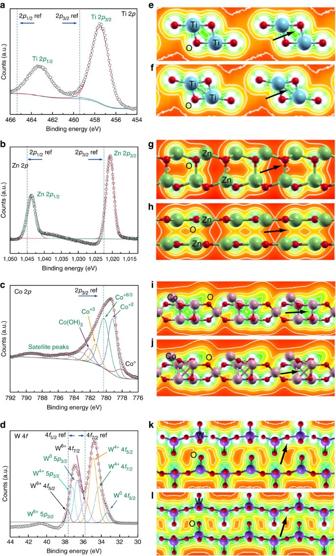Figure 3: Surface chemical states of 2D transition metal oxide nanosheets. (a–d) XPS spectra of the ultrathin 2D metal oxide nanosheets: (a) TiO2, (b) ZnO, (c) Co3O4and (d) WO3, where the binding energies show 0.5–2 eV shifting to the low binding energy range compared with the corresponding bulk material surface states; (e,f) atomic structures and slices of the total charge density distribution in the (010) plane of bulk anatase TiO2(e) and the TiO22D monolayer nanosheets (f), showing the redistribution of electron densities and the extra bonding formed between Ti–Ti in the TiO22D nanosheets; (g,h) atomic structures and slices of the total charge density distribution in the (001) plane of bulk wurtzite ZnO (g) and the ZnO 2D bilayer nanosheets (h), showing the redistribution of electron densities and the interlayer bond breaking between Zn–O–Zn in the ZnO 2D nanosheets; (i,j) atomic structures and slices of the total charge density distribution in the (010) plane of bulk Co3O4(i) and the Co3O42D monolayer nanosheets (j), showing the redistribution of electron densities and the extra bonding formed between Co–Co in the Co3O42D nanosheet; (k,l) atomic structures and slices of the total charge density distribution in the (100) plane of bulk monoclinic WO3(k) and the WO32D bilayer nanosheets (l), showing the redistribution of electron densities and the crystal structure distortion in the WO32D nanosheets. The arrows in (e–l) indicate the structural differences between the ultrathin 2D nanosheets and the corresponding bulk inner atoms: new bond formation between Ti–Ti (e,f), bond breaking between Zn–O (g,h), new bond formation between Co–Co (i,j) and bond distortion between W–O (k,l). Figure 3: Surface chemical states of 2D transition metal oxide nanosheets. ( a – d ) XPS spectra of the ultrathin 2D metal oxide nanosheets: ( a ) TiO 2 , ( b ) ZnO, ( c ) Co 3 O 4 and ( d ) WO 3 , where the binding energies show 0.5–2 eV shifting to the low binding energy range compared with the corresponding bulk material surface states; ( e , f ) atomic structures and slices of the total charge density distribution in the (010) plane of bulk anatase TiO 2 ( e ) and the TiO 2 2D monolayer nanosheets ( f ), showing the redistribution of electron densities and the extra bonding formed between Ti–Ti in the TiO 2 2D nanosheets; ( g , h ) atomic structures and slices of the total charge density distribution in the (001) plane of bulk wurtzite ZnO ( g ) and the ZnO 2D bilayer nanosheets ( h ), showing the redistribution of electron densities and the interlayer bond breaking between Zn–O–Zn in the ZnO 2D nanosheets; ( i , j ) atomic structures and slices of the total charge density distribution in the (010) plane of bulk Co 3 O 4 ( i ) and the Co 3 O 4 2D monolayer nanosheets ( j ), showing the redistribution of electron densities and the extra bonding formed between Co–Co in the Co 3 O 4 2D nanosheet; ( k , l ) atomic structures and slices of the total charge density distribution in the (100) plane of bulk monoclinic WO 3 ( k ) and the WO 3 2D bilayer nanosheets ( l ), showing the redistribution of electron densities and the crystal structure distortion in the WO 3 2D nanosheets. The arrows in ( e – l ) indicate the structural differences between the ultrathin 2D nanosheets and the corresponding bulk inner atoms: new bond formation between Ti–Ti ( e , f ), bond breaking between Zn–O ( g , h ), new bond formation between Co–Co ( i , j ) and bond distortion between W–O ( k , l ). Full size image Table 1 Electron charge distribution of the 2D transition metal oxide nanosheets and the corresponding bulk materials as quantified by Löwdin atomic populations. Full size table It is interesting that some ultrathin 2D TiO 2 nanosheets present unusual exposed facets. Lattice images of the anatase ultrathin TiO 2 2D nanosheets can be seen in Supplementary Fig. 2d . By combining the selected area electron diffraction patterns with the HRTEM images ( Supplementary Fig. 2c ), it is easy to determine that the exposed surfaces of the anatase TiO 2 nanosheets are high-energy {010} facets. It has been demonstrated that exposed high-energy surfaces are crucial for improving the chemical activity of TiO 2 (refs 34 , 35 ). Although the surface energy of anatase {010} (0.53 J m −2 ) was calculated to be between those of {001} (0.90 J m −2 ) and {101} (0.44 J m −2 ), no {010} appears in the equilibrium shape of anatase crystals or nanostructures [35] . The presence of the high percentage of exposed high-energy anatase {010} surfaces in the ultrathin 2D TiO 2 nanosheets would endow them with high chemical activity [35] . For the exposed surfaces of ZnO, Co 3 O 4 and WO 3 , however, no such high-energy exposed surfaces were observed. It is certain that the special shapes and electronic structures will induce some salient properties in the ultrathin 2D nanosheets. One of the most obvious features is the high specific surface area ( Supplementary Fig. 14 ). An enhancement of the specific surface area by 3–10 times compared with nanoparticles prepared via the conventional synthesis strategies is achieved. The ultrathin TiO 2 nanosheets exhibit an ultrahigh specific surface area of 298 m 2 g −1 , which is almost sixfold higher than that of the commercial P25 TiO 2 nanoparticles ( ∼ 50 m 2 g −1 ). Besides the high surface area of 2D TiO 2 nanosheets, the specific surface area of the ZnO 2D nanosheets is up to 265 m 2 g −1 , the Co 3 O 4 2D nanosheets of 246 m 2 g −1 and the WO 3 2D nanosheets of 157 m 2 g −1 . It is known that the higher the specific surface area is, the larger the amount of active reaction sites on the surface. The high specific surface areas of the 2D metal oxide nanosheets would guarantee their high chemical reaction activity. Another feature is the shifting in the band structure aroused by the confinement, which is due to the atomic scale thickness of the nanosheets. All the ultraviolet–visible (UV–vis) adsorption spectra of the TiO 2 , ZnO, Co 3 O 4 and WO 3 nanosheets ( Supplementary Fig. 12 ) show an obvious blue shift compared with the bulk materials, demonstrating their significant quantum confinement effect in the thinnest dimension. It is a general understanding that smaller size of transitional metal oxide nanoparticles raises the conduction band and lowers the valence band, and results in the observation of a blue shift in the absorption edge, or we called quantum size effect. On the basis of the study by Saton et al. [36] , however, the significant quantum size effect can only be observed for the nanoparticles with diameters <2 nm, in the case of TiO 2 . The commonly used transitional metal oxide nanoparticles usually have diameters much larger than 2 nm. For example, one of the typical TiO 2 nanoparticles, P25, has an average diameter of 20 nm. In the present work, the thicknesses of the ultrathin 2D nanosheets were in the range of 1.5–5.2 nm in the form of stacks and below 1 nm for monolayers, which are in the range for the size with significant quantum size effect. Thus, these ultrathin 2D nanosheets would have much more significant quantum size effect than those of the normally used nanoparticles. Owing to the high surface area, chemically active exposed surface and confined thickness, it is expected that these unique ultrathin 2D nanosheets would be attractive in a variety of applications, from nanostructured electronic or photonic devices to energy generation and storage systems. Performance of transparent and flexible ultraviolet photodetectors To explore the applicability of 2D nanostructures, we examined the performance of transparent, flexible ultraviolet (UV) photodetectors by depositing the ultrathin 2D metal oxide nanosheets on a single-layer graphene back electrode ( Fig. 4 ). Visible-light-blind ultraviolet (UV-A band at 320–400 nm) photodetectors have attracted intensive interest for their wide applications in healthcare, climate control, agriculture, astronomy and aeronautics [37] . The ultrathin 2D metal oxide nanosheets prepared in the present work feature widened bandgaps, which allow the transmission of visible light but high responses to ultraviolet light, and are the most promising candidates for high-performance ultraviolet photodetectors. 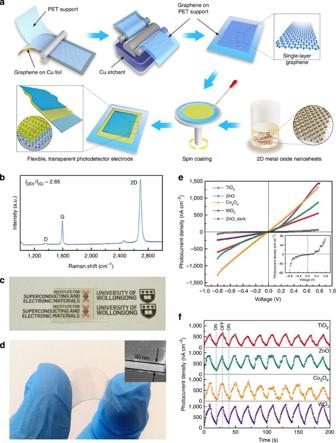Figure 4: Fabrication and performance of transparent and flexible 2D nanosheet photodetector. (a) Schematic diagram of the fabrication of the photodetector electrode, consisting of one single-layer graphene sheet on PET substrate and a thin layer of spin-coated 2D metal oxide nanosheets; (b) Raman spectrum of the as-prepared graphene on PET film, demonstrating the single-layer feature, where the 2D-band is much more intense and sharper compared with the 2D-band in multilayer graphene, and with an intensity ratio of 2D/G peaks of around 2.65 (ref. 41)41; (c) the fabricated 2D nanosheet layers on the graphene-PET photodetector electrode show its high transparency and (d) flexibility, with the inset containing an SEM cross-section image of the photoelectrode indshowing that the thickness of the deposited 2D metal oxide nanosheets on the single-layer graphene-PET substrate was around 50 nm; (e)I–Vcharacteristics of the transparent, flexible photodetector devices constructed from the 2D nanosheets of TiO2, ZnO, Co3O4and WO3, respectively, under 325 nm ultraviolet light (67 mW cm−2) irradiation, with the inset presenting theI–Vcharacteristic of the dark photocurrent of the ZnO 2D nanosheet photoanode; and (f) the photoresponse behaviour of the transparent, flexible photodetectors under alternating on and off 325 nm ultraviolet light (67 mW cm−2), with an interval of 10 s and a bias of 0.5 V. Figure 4: Fabrication and performance of transparent and flexible 2D nanosheet photodetector. ( a ) Schematic diagram of the fabrication of the photodetector electrode, consisting of one single-layer graphene sheet on PET substrate and a thin layer of spin-coated 2D metal oxide nanosheets; ( b ) Raman spectrum of the as-prepared graphene on PET film, demonstrating the single-layer feature, where the 2D-band is much more intense and sharper compared with the 2D-band in multilayer graphene, and with an intensity ratio of 2D/G peaks of around 2.65 (ref. 41) [41] ; ( c ) the fabricated 2D nanosheet layers on the graphene-PET photodetector electrode show its high transparency and ( d ) flexibility, with the inset containing an SEM cross-section image of the photoelectrode in d showing that the thickness of the deposited 2D metal oxide nanosheets on the single-layer graphene-PET substrate was around 50 nm; ( e ) I – V characteristics of the transparent, flexible photodetector devices constructed from the 2D nanosheets of TiO 2 , ZnO, Co 3 O 4 and WO 3 , respectively, under 325 nm ultraviolet light (67 mW cm −2 ) irradiation, with the inset presenting the I – V characteristic of the dark photocurrent of the ZnO 2D nanosheet photoanode; and ( f ) the photoresponse behaviour of the transparent, flexible photodetectors under alternating on and off 325 nm ultraviolet light (67 mW cm −2 ), with an interval of 10 s and a bias of 0.5 V. Full size image Figure 4 shows the preparation of the single-layer graphene back electrode for the photodetector, deposition of ultrathin 2D transition metal oxide nanosheets on the single-layer graphene and the performance of the transparent, flexible ultraviolet photodetector. As schematically illustrated in Fig. 4a , the single-layer graphene on the 188-μm thick polyethylene terephthalate (PET) substrate was prepared by transferring the chemical vapour-deposited graphene on Cu foil to PET via a roll-to-roll production method described elsewhere [38] , [39] , [40] . The Raman spectrum clearly proves that the obtained graphene is single layer ( Fig. 4b ), based on the method to determine the number of layers of graphene from the 2D-band, as the intensity ratio of the 2D-band to the G-band is ∼ 2.65 (ref. 41) [41] . Then, well-dispersed diluted ultrathin 2D metal oxide nanosheets in ethanol suspensions were spin-coated onto the graphene substrate to form a transparent and flexible photoelectrode ( Fig. 4c,d ). To ensure significant signal intensities in the photoelectrode, the thickness of the deposited 2D metal oxide nanosheet layer was kept at around 50 nm. After assembly with a graphene-PET counter electrode, the transparent, flexible ultraviolet photodetectors were tested under 325 nm ultraviolet light (67 mW cm −2 ) or an alternating on and off ultraviolet source with an interval of 10 s. Figure 4e presents the I – V characteristics of the transparent, flexible ultraviolet photodetectors. The photocurrent densities of the photodetectors made from the 2D transition metal oxide nanosheets reach the order of mA cm −2 . Except for the WO 3 photodetector, which presents an obvious p -type Schottky barrier contact, the others show ideal linear I – V responses under the ultraviolet irradiation and good ohmic behaviours. The linear I – V response, or the ohmic behaviour, is very desirable because it enhances the photosensitive properties of the devices. The I – V characteristics demonstrate that the TiO 2 , ZnO and Co 3 O 4 2D ultrathin nanosheets are promising candidates due to their ohmic behaviour and the large output signal. Figure 4f shows the photoresponses of the ultraviolet photodetectors under the alternating on and off ultraviolet light with an interval of 10 s and a bias of 0.5 V. All of the time responses of the devices are highly stable and reproducible. No degradation was found in tens of on–off switching cycles, confirming the excellent stability and fast response speed of our device. It is interesting that the WO 3 photoelectrodes presented increasing photocurrents with prolonged irradiation time, due to its photochromic effect under ultraviolet irradiation [42] . These findings show the promising potential of these ultrathin 2D metal oxide nanostructures for practical applications such as photoelectric or photochemical devices. In this work, we demonstrate that the generalized bottom-up synthetic method for ultrathin 2D transition metal oxide nanosheets is of great interest for making various functional nanostructures with high surface area, high chemical activity and a quantum confinement effect. Such unique ultrathin 2D nanostructures could be the fundamental basis for emerging applications in not only energy generation/storage systems, but also electronic devices and sensors. Moreover, this kind of nanostructure may also provide unique mechanical, thermal and anti-corrosive properties that would be useful in transparent protective coatings, barrier films and reinforcement materials. Synthesis of ultrathin 2D TiO 2 nanosheets Titanium isopropoxide (TTIP, 1.05 g) was added into 0.74 g concentrated HCl solution during vigorous stirring (bottle A); and 0.2 g polyethylene oxide–polypropylene oxide–polyethylene oxide (PEO 20 –PPO 70 –PEO 20 , Pluronic P123) was dissolved in 3.0 g ethanol (EtOH) (bottle B). After stirring for 15 min, the solution in bottle B was added into bottle A and stirred for another 30 min. Then, 2.5 ml TTIP solution with 20 ml EG was transferred into a 45-ml autoclave and heated at 150 °C for 20 h. The products of the hydrothermal reaction were washed with ethanol three times, and the white powders were collected after washing/centrifugation and drying at 80 °C for 24 h. Synthesis of ultrathin 2D ZnO nanosheets Pluronic P123 (0.2 g) was added into 3 g EtOH with 0.45 g H 2 O to form a clear solution with stirring for 15 min, and then 0.1 g ZnAc 2 ·2H 2 O and 0.045 g hexamethylenetetramine (HMTA) were added into the ethanol solution. After stirring for around 15 min, a clear solution was obtained. Then, 46 ml EG was added into the ethanol solution. After stirring for 30 min, a transparent solution was obtained. The obtained EtOH+EG precursor solution was statically aged for 7 days. After aging, the transparent precursor solution was divided into two parts, transferred into two 45 ml autoclaves and heated at 110 °C for 15 h. The products of the solvothermal reaction were washed with distilled water and ethanol three times, and the light yellow powders were collected after washing/centrifugation and drying at 80 °C for 24 h. Synthesis of ultrathin 2D Co 3 O 4 nanosheets Pluronic P123 (0.2 g) was added into 13 g EtOH with 1 g H 2 O to form a clear solution with stirring for 15 min, and then 0.125 g Co(Ac) 2 ·4H 2 O and 0.07 g HMTA were added into the ethanol solution. After stirring for around 15 min, a purple solution was obtained. Then, 13 ml EG was added into the ethanol solution. After stirring for 30 min, a transparent solution was obtained. The obtained EtOH+EG precursor solution was statically aged for 1 day. After aging, the transparent precursor solution was transferred into a 45 ml autoclave and heated at 170 °C for 2 h. The products of the solvothermal reaction were washed with distilled water and ethanol three times, and the brown powders were collected after washing/centrifugation and dehydration at 150–400 °C for 2 h. Synthesis of ultrathin 2D WO 3 nanosheets Pluronic P123 (0.2 g) was added into 13 g EtOH with 0.45 g H 2 O to form a clear solution with stirring for 15 min, and then 0.4 g WCl 6 was added into the ethanol solution. After stirring for around 15 min, a yellow solution was obtained. Then, the precursor solution was transferred into a 45 ml autoclave and heated at 110 °C for 2 h. The products of the solvothermal reaction were washed with ethanol three times, and the white-blue powders were collected after washing/centrifugation and drying at 80 °C for 24 h. Characterization The composition and phase of the as-prepared products were evaluated using a powder X-ray diffractometer (XRD, MMA, GBC Scientific Equipment LLC, Hampshire, IL, USA) with Cu Kα radiation. The chemical states of the nanostructures were determined by XPS (PHOIBOS 100 Analyser from SPECS; Al K α X-rays, Berlin, Germany). The morphology of the samples was observed with a SEM (JSM-7500FA, JEOL, Tokyo, Japan). HRTEM observation was carried out using a JEM-2011F (JEOL) operated at 200 kV. The thickness of the 2D ultrathin nanosheets was determined by AFM (MPF-3D, Asylum Research, Santa Barbara, USA). For AFM observation, a nanosheet specimen was prepared by quickly dipping single-crystal silicon substrate with a 100-nm-thick amorphous SiO 2 top layer into diluted acetone-dispersed 2D metal oxide nanosheet solution. Surface area was measured by a surface area analyzer (NOVA1000, Quantachrome Co., FL, USA) at 77 K. Before the measurement, the sample was heated at 120 °C for 5 h. Photocurrent performance tests Single-layer graphene on 188-μm thick PET substrate was prepared by transferring chemical vapour-deposited graphene on Cu foil to PET based a roll-to-roll production method described elsewhere [38] , [39] , [40] . Briefly, coarse-grain copper foil was heated to 1,000 °C, and then a flowing gas mixture of CH 4 and H 2 was introduced at 460 mtorr and 8 sccm for 30 min, followed by rapid cooling to room temperature under flowing H 2 . The graphene grown on copper foil was attached to a 188-μm thick PET supporting film and passed through two heated rollers for soft pressing. After removing the copper substrate by electrochemical reaction with aqueous 0.1 M ammonium persulphate solution (NH 4 ) 2 S 2 O 8 , the single-layer graphene was transferred onto the PET supporting film. Transparent, flexible photoelectrode was prepared by spin-coating techniques. A well-dispersed, 0.1 mg ml −1 2D transition metal oxide nanosheet ethanol solution was dropped onto sliced, single-layer, graphene-PET substrate and spin-coated at 2,000 r.p.m. for 30 s. To reach the target thickness, 2–5 repetitions of the coating process were needed. The coated photoelectrodes were then aged in covered petri dishes at room temperature for 24 h. After aging, the photoelectrodes were dried at 80 °C for 12 h. A photosensitive detector was fabricated by attaching the photoelectrode made from 2D metal oxide nanosheets with another uncoated flexible single-layer graphene-PET counter electrode. The photocurrent was examined by a Keithley 2400 source meter under a 325-nm ultraviolet (UV) light source (67 mW cm −2 ) or an alternating on and off ultraviolet source (67 mW cm −2 ) with an interval of 10 s. DFT calculations The first-principle calculations were carried out within the framework of spin-polarized plane-wave DFT, implemented in the Quantum-Espresso package [43] . The Perdew–Burke–Ernzerhof variant of the generalized gradient approximation was used for the exchange-correlation potential [44] . The valence-ion interaction was described by ultrasoft pseudopotentials [45] . A plane-wave cutoff energy of 40 Ry was adopted for the plane-wave expansion of the wave function to converge the relevant quantities. For Brillouin-zone integrations, a Monkhorst-Pack mesh [46] of 5 × 5 × 1 k -points was used for structural optimization, while a denser mesh of 15 × 15 × 1 was used for electronic structure analysis. In our calculations, TiO 2 , ZnO, Co 3 O 4 and WO 3 nanosheets have been described using supercells, respectively, by monolayer TiO 2 sheets parallel to (010), bilayer ZnO sheets parallel to (001), monolayer Co 3 O 4 sheets parallel to (001) and bilayer WO 3 sheets parallel to (100). A large vacuum spacing of 15 Å between 2D nanosheets was selected to prevent spurious interactions between the periodic layers. All atomic positions and lattice constants were optimized by using the Broyden–Fletcher–Goldfarb–Shanno algorithm [47] . The convergence for the residual forces is <10 −3 Ry per Bohr (2.6 × 10 −2 eV Å −1 ) on ionic relaxation. How to cite this article: Sun, Z. et al. Generalized self-assembly of scalable two-dimensional transition metal oxide nanosheets. Nat. Commun. 5:3813 doi: 10.1038/ncomms4813 (2014).